Acquisition of aluminium tolerance by modification of a single gene in barley Originating from the Fertile Crescent in the Middle East, barley has now been cultivated widely on different soil types including acid soils, where aluminium toxicity is a major limiting factor. Here we show that the adaptation of barley to acid soils is achieved by the modification of a single gene ( HvAACT1 ) encoding a citrate transporter. We find that the primary function of this protein is to release citrate from the root pericycle cells to the xylem to facilitate the translocation of iron from roots to shoots. However, a 1-kb insertion in the upstream of the HvAACT1 coding region occurring only in the Al-tolerant accessions, enhances its expression and alters the location of expression to the root tips. The altered HvAACT1 has an important role in detoxifying aluminium by secreting citrate to the rhizosphere. Thus, the insertion of a 1-kb sequence in the HvAACT1 upstream enables barley to adapt to acidic soils. Aluminium (Al) and iron (Fe) are the two most abundant metals in the Earth's crust. The two metals have contrasting effects on plant growth; aluminium is a toxic metal, whereas iron is essential for plant growth. Therefore, plants rooting in soils must employ strategies to acquire iron, but to detoxify aluminium. Plants have developed two distinct strategies for the acquisition of iron from the soil [1] . The first strategy is employed by dicotyledonous and non-gramineous monocotyledonous species, and is characterized by the release of proton (H + ) and reductants/chelators (for example, electron (e), organic acids and phenolics) into the rhizosphere, thereby increasing iron solubility [1] . By contrast, Fe-acquisition by the second strategy, which is employed only by gramineous species, involves the secretion of hexadentate Fe 3+ -chelating substances (phytosiderophores as mugineic acids) and subsequent uptake of Fe 3+ chelates [2] . Most of the genes responsible for the different steps of iron acquisition have been isolated [1] . In contrast to Fe, aluminium is not essential to plants. Although metallic aluminium and aluminosilicate minerals are nontoxic, ionic aluminium (mainly Al 3+ ), which is released into the soil under acidic conditions, is toxic to all living cells. This form of Al rapidly inhibits root elongation at the micromolar level by targeting multiple cellular sites, including the cell wall and the plasma membrane, and various cellular processes, such as signal transduction pathways and calcium homeostasis [3] , [4] . Consequently, aluminium inhibits the uptake of water and nutrients and increases the sensitivity of plants to various stresses, especially drought. Aluminium toxicity has, therefore, been recognized as a major factor limiting crop production on acid soils, which comprise 30–40% of arable soils in the world [5] . However, some plant species or accessions have evolved strategies to cope with Al toxicity [6] , [7] , [8] . One of the most common mechanisms is the secretion of organic acid anions, such as citrate, oxalate and malate, from the roots [9] , [10] , [11] . These organic acid anions are able to chelate Al in the rhizosphere, thus preventing Al from binding to the root cell components [9] . Many plant species including both dicots and monocots are known to adopt this mechanism [9] , [10] , [11] . Genes encoding transporters for the Al-induced secretion of malate and citrate have been identified. The malate transporter gene ALMT1 was isolated in wheat and Arabidopsis [12] , [13] . Genes responsible for the Al-induced citrate secretion have also been identified in barley, sorghum, and other plant species [14] , [15] , [16] , [17] , [18] , [19] . Barley ( Hordeum vulgare ), the fourth most important cereal crop for human food and animal feed, is one of the most Al-sensitive species among the small grain cereals; however, there is a wide variation in Al tolerance among barley cultivars [20] . This variation has been found to correlate with the amount of citrate secretion from the roots [20] . Furthermore, the Al-induced secretion of citrate from barley roots is mediated by HvAACT1 (Al-activated citrate transporter 1) [14] , which is a member of the multidrug and toxic compound extrusion (MATE) family. HvAACT1 is localized to the plasma membrane of the root epidermal cells [14] . Although the expression of HvAACT1 is not induced by Al, its expression level is constitutively higher in the Al-tolerant cultivars consistent with greater citrate secretion [14] . However, the mechanisms underlying the different expressions of HvAACT1 in different barley cultivars are unknown. Here we report that a 1-kb insertion in the upstream enhances the expression of HvAACT1 in the Al-tolerant cultivars. Furthermore, we found that this insertion also alters the spatial expression of HvAACT1 from the original location in the mature root zone (required for the root-to-shoot translocation of iron) to the root tips, which are the sensitive targets of Al toxicity. Evolutional analysis showed that the insertion occurs only in the Al-tolerant cultivars from Japan, Korea and China, a result of adaptation to the acid soils in these areas. Comparison of the HvAACT1 genome sequence We have previously shown that the Al-sensitive barley cultivar Morex and the Al-tolerant cultivar Murasakimochi differed in the level of HcAACT1 expression [14] . To investigate the underlying mechanism, we analysed the genome sequences of HvAACT1 in both cultivars. We found an insertion with 1,023 bp in the upstream of HvAACT1 coding region in Murasakimochi, but not in Morex ( Fig. 1a , Supplementary Fig. S1 ). HvAACT1 is characterized by a large intron (about 6 kb) in the 5′-untranslated region (UTR) region and this insertion is localized at 4.8 kb upstream from initiating codon (ATG) in the Murasakimochi genome ( Fig. 1a , Supplementary Fig. S1 ). We then checked this insertion in other cultivars and found that it is present in all Al-tolerant cultivars tested ( Fig. 1b ). Database search revealed that the insertion shows similarity with the CACTA-like transposon in rice. Furthermore, this insertion has a terminal inverted repeats (17 bp) at the 5′ end and 3′ end ( Fig. 1c ). 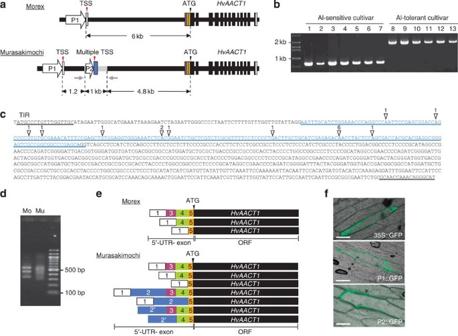Figure 1: Location and function of the upstream insertion. (a) Schematic presentation of the genomic structure ofHvAACT1in an Al-sensitive cultivar (Morex; Mo) and an Al-tolerant cultivar (Murasakimochi; Mu). White and colour vertical boxes show UTR exons. Black vertical boxes and black lines show ORF-exons and introns, respectively. Grey line shows a 1,023-bp insertion at the 4.8 kb upstream of the coding region in Murasakimochi. TSS, transcriptional start site. Grey arrows indicate the positions of PCR primers used for the insertion detection inb. (b) Detection of the 1-kb upstream insertion in different barley cultivars. 1, Morex; 2, Golden Promise; 3, BC95; 4, Z504; 5, K0046; 6, BC282; 7, BC366; 8, ALP3; 9, BC26; 10, Murasakimochi; 11, BC262; 12, BC191; 13, Akashinriki. (c) Sequence ofHvAACT1upstream insertion. White triangles show multipleHvAACT1TSS and the number means frequency of identification of TSS by cloning. Sequence of blue character indicates 5′-UTR-2 in Murasakimochi. The insertion region contains a terminal inverted repeat (TIR) of 17 bp at the 5′ and 3′ ends. (d) Image of agarose gel showing the 5′-RACE PCR products.HvAACT1gene-specific primer and RNA oligo primer were used for amplifying HvAACT1 5′-UTR region. (e) Schematic presentation of 5′-UTR variants ofHvAACT1between Morex and Murasakimochi. The sequences were read from 20 5′-RACE clones. White and colour boxes show the 5′-UTR and colours corresponding to diagram ina. The number in the box shows 5′-UTR position on the genome. Box 2′ includes variations from different transcriptional start sites. (f) Promoter assay. Common promoter (P1 ina), 1-kb insertion-originated region (P2 ina), or 35S promoter (as a control) was fused to GFP and then transiently introduced to onion epidermal cells. Scale bars, 100 μm. Figure 1: Location and function of the upstream insertion. ( a ) Schematic presentation of the genomic structure of HvAACT1 in an Al-sensitive cultivar (Morex; Mo) and an Al-tolerant cultivar (Murasakimochi; Mu). White and colour vertical boxes show UTR exons. Black vertical boxes and black lines show ORF-exons and introns, respectively. Grey line shows a 1,023-bp insertion at the 4.8 kb upstream of the coding region in Murasakimochi. TSS, transcriptional start site. Grey arrows indicate the positions of PCR primers used for the insertion detection in b . ( b ) Detection of the 1-kb upstream insertion in different barley cultivars. 1, Morex; 2, Golden Promise; 3, BC95; 4, Z504; 5, K0046; 6, BC282; 7, BC366; 8, ALP3; 9, BC26; 10, Murasakimochi; 11, BC262; 12, BC191; 13, Akashinriki. ( c ) Sequence of HvAACT1 upstream insertion. White triangles show multiple HvAACT1 TSS and the number means frequency of identification of TSS by cloning. Sequence of blue character indicates 5′-UTR-2 in Murasakimochi. The insertion region contains a terminal inverted repeat (TIR) of 17 bp at the 5′ and 3′ ends. ( d ) Image of agarose gel showing the 5′-RACE PCR products. HvAACT1 gene-specific primer and RNA oligo primer were used for amplifying HvAACT1 5′-UTR region. ( e ) Schematic presentation of 5′-UTR variants of HvAACT1 between Morex and Murasakimochi. The sequences were read from 20 5′-RACE clones. White and colour boxes show the 5′-UTR and colours corresponding to diagram in a . The number in the box shows 5′-UTR position on the genome. Box 2′ includes variations from different transcriptional start sites. ( f ) Promoter assay. Common promoter (P1 in a ), 1-kb insertion-originated region (P2 in a ), or 35S promoter (as a control) was fused to GFP and then transiently introduced to onion epidermal cells. Scale bars, 100 μm. Full size image Determination of the transcriptional start sites We determined the potential transcriptional start sites of HvAACT1 using 5′-RACE. Although there were three different 5′-UTR sequences in Morex, there was only one transcriptional start site (TSS) at 6 kb upstream from ATG of HvAACT1 ( Fig. 1d,e ). By contrast, there were multiple TSSs in Murasakimochi in addition to the same TSS found in Morex. These TSSs originated from the insertion ( Fig. 1c ), yielding various mRNAs with different 5′-UTR during splicing processes ( Fig. 1d,e ). In addition, these 5′-UTR sequences did not contain an initiating codon. All transcripts encode the same functional gene ( Fig. 1e ). Promoter activity assay To investigate the function of this insertion, we determined the promoter activity by transiently introducing green fluorescent protein (GFP) fused with a part (262 bp) of the insertion before most TSSs into onion epidermal cells. A putative common promoter and the 35S promoter were also fused with GFP for comparison. GFP signal was observed in the cells introducing all promoters ( Fig. 1f ). These results indicate that the insertion functions as a promoter in onion epidermal cells. Expression patterns To investigate how this additional promoter in the insertion region affects the expression of HvAACT1 , we performed a detailed expression analysis of the 5′-UTR region. The HvAACT1 expression level gradually increased behind the multiple TSS sites ( Fig. 2 ). Spatial analysis showed that the expression level at the common UTR was very low in the root tips (0–3 mm) of both Murasakimochi and Morex ( Fig. 3a–c ). In the other parts of the roots, the expression level at the common UTR in Morex was slightly higher than or similar to that of Murasakimochi. At the insertion-specific region, the expression was detected only in Murasakimochi, with both the root tips (0–3 mm) and the other parts of roots showing similar levels of expression ( Fig. 3c ). For the coding region, the expression level was 50 times higher in Murasakimochi than in Morex in the root tips and 3 times higher in the other parts of roots ( Fig. 3c ). 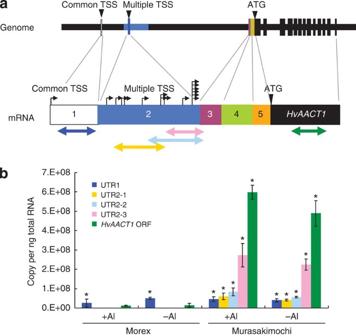Figure 2:HvAACT1expression level at different 5′-UTR regions. (a) A schematic model of primer position and gene structure. The colour arrows show regions for PCR amplification inb. Black arrows show TSS. (b)HvAACT1expression at different 5′-UTR region. The colour of column corresponds to that ina. Statistical comparison was performed by one-way ANOVA followed by Dunnett's multiple comparison test. All data were compared with the expression of Morex ORF in the –Al treatment. *P<0.05. Data are shown as the mean values±s.d. (n=3). Figure 2: HvAACT1 expression level at different 5′-UTR regions. ( a ) A schematic model of primer position and gene structure. The colour arrows show regions for PCR amplification in b . Black arrows show TSS. ( b ) HvAACT1 expression at different 5′-UTR region. The colour of column corresponds to that in a . Statistical comparison was performed by one-way ANOVA followed by Dunnett's multiple comparison test. All data were compared with the expression of Morex ORF in the –Al treatment. * P <0.05. Data are shown as the mean values±s.d. ( n =3). 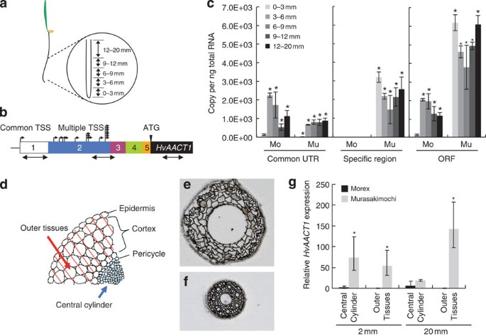Figure 3: Altered expression patterns ofHvAACT1by a 1-kb upstream insertion. (a) Schematic presentation of sampling position of roots. (b) Primer location designed for spatial expression analysis. The white and colour boxes showed 5′-UTR sequences of Morex (Mo) and Murasakimochi (Mu). Small black arrows show TSS. Large black arrows show regions for PCR amplification. The number in the boxes shows the position of 5′-UTR. (c) Spatial expression ofHvAACT1in different root zones assayed with different primer sets at the common 5′-UTR, the insertion region and the coding region ofHvAACT1, respectively, as shown inb. (d) Schematic presentation of different tissue samples separated by laser microdissection. The epidermis and cortex were collected as outer tissues and inner tissues from pericycle as central cylinder. (e,f) Outer tissues (e) and central cylinder (f) of the roots after laser microdissection. (g) Tissue-specific expression ofHvAACT1. Expression level relative to 2 mm central cylinder of Morex is shown. Data incandgare shown as the mean values±s.d. (n=3). Statistical comparison was performed by one-way ANOVA followed by Dunnett's multiple comparison test. (c) All data were compared with 0–3 mm Morex assayed with the ORF primer. *P<0.05. (g) The expression was compared with the central cylinder of Morex at 20 mm. *P<0.05. Full size image Figure 3: Altered expression patterns of HvAACT1 by a 1-kb upstream insertion. ( a ) Schematic presentation of sampling position of roots. ( b ) Primer location designed for spatial expression analysis. The white and colour boxes showed 5′-UTR sequences of Morex (Mo) and Murasakimochi (Mu). Small black arrows show TSS. Large black arrows show regions for PCR amplification. The number in the boxes shows the position of 5′-UTR. ( c ) Spatial expression of HvAACT1 in different root zones assayed with different primer sets at the common 5′-UTR, the insertion region and the coding region of HvAACT1 , respectively, as shown in b . ( d ) Schematic presentation of different tissue samples separated by laser microdissection. The epidermis and cortex were collected as outer tissues and inner tissues from pericycle as central cylinder. ( e , f ) Outer tissues ( e ) and central cylinder ( f ) of the roots after laser microdissection. ( g ) Tissue-specific expression of HvAACT1 . Expression level relative to 2 mm central cylinder of Morex is shown. Data in c and g are shown as the mean values±s.d. ( n =3). Statistical comparison was performed by one-way ANOVA followed by Dunnett's multiple comparison test. ( c ) All data were compared with 0–3 mm Morex assayed with the ORF primer. * P <0.05. ( g ) The expression was compared with the central cylinder of Morex at 20 mm. * P <0.05. Full size image Tissue-specific expression of HvAACT1 To examine the tissue-specific expression of HvAACT1 , we obtained RNA from the central cylinder (pericycle and inner tissues) and the outer tissues (cortex and epidermis) of root tissues by using laser microdissection ( Fig. 3d–f ). In the root tips (around 2 mm from the apex), the expression of HvAACT1 was hardly detected in either the central cylinder or the outer tissues of Morex ( Fig. 3g ). By contrast, HvAACT1 was expressed at a higher level in both tissues in Murasakimochi ( Fig. 3g ). In the mature zone (around 20 mm from the apex) where xylem is well developed, the expression level of HvAACT1 in the central cylinder was similar between Morex and Murasakimochi ( Fig. 3g ). However, in the outer tissues, no expression of HvAACT1 was detected in Morex, whereas a high expression was found in Murasakimochi. Transformation of HvAACT1 into barley To further investigate the role of the 1-kb insertion in Al tolerance, we introduced HvAACT1 into an Al-sensitive cultivar (Golden Promise) under the control of three different promoters; the specific insertion region (B3), promoters of Murasakimochi (B1) or Morex (B2) ( Supplementary Fig. S2 ). Analysis with T0 plants showed that there was a positive correlation between the HvAACT1 expression level and citrate secretion in transgenic plants carrying the Murasakimochi promoter (B1) and the specific insertion region (B3; Supplementary Fig. S3 ). We randomly selected four independent lines for further analysis. In the T1 transgenic lines, the expression level of HvAACT1 in the root tips (0–3 mm) was significantly enhanced in the lines carrying HvAACT1 driven by the Murasakimochi promoter or the specific insertion region ( Fig. 4a,d ), but was unaffected in those carrying the Morex promoter. Similarly, Al-induced secretion of citrate and Al tolerance were significantly enhanced in the lines driven by the Murasakimochi promoter or the insertion region ( Fig. 4b,c,e,f ), but not in those driven by the Morex promoter. These results indicate that the specific insertion enhances the expression of HvAACT1 in the root tips, resulting in enhanced Al-induced secretion of citrate and subsequently Al tolerance. 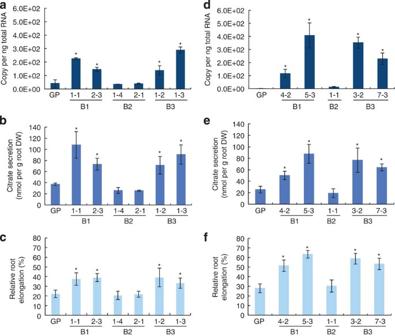Figure 4: Function of the upstream insertion in transgenic barley. (a) Expression ofHvAACT1in the root tips (0–3 mm). Plasmids containingHvAACT1ORF fused with Murasakimochi promoter (B1), Morex promoter (B2) or insertion-originated promoter (B3) were transformed into the barley cultivar Golden Promise (GP). (b) Al-induced secretion of citrate. (c) Al tolerance in transgenic barley lines. (d–f) Expression ofHvAACT1in the root tips (0–3 mm) (d), Al-induced secretion of citrate (e) and Al tolerance in transgenic barley lines (f) in a separate experiment using different independent lines. Data are shown as the means±s.d. (n=3) fora,b,d,eand (n=10) forc,f. Statistical comparison was performed by one-way ANOVA followed by the Tukey's multiple comparison test. All data were compared with GP. *P<0.05. Figure 4: Function of the upstream insertion in transgenic barley. ( a ) Expression of HvAACT1 in the root tips (0–3 mm). Plasmids containing HvAACT1 ORF fused with Murasakimochi promoter (B1), Morex promoter (B2) or insertion-originated promoter (B3) were transformed into the barley cultivar Golden Promise (GP). ( b ) Al-induced secretion of citrate. ( c ) Al tolerance in transgenic barley lines. ( d – f ) Expression of HvAACT1 in the root tips (0–3 mm) ( d ), Al-induced secretion of citrate ( e ) and Al tolerance in transgenic barley lines ( f ) in a separate experiment using different independent lines. Data are shown as the means±s.d. ( n =3) for a , b , d , e and ( n =10) for c , f . Statistical comparison was performed by one-way ANOVA followed by the Tukey's multiple comparison test. All data were compared with GP. * P <0.05. Full size image Role of HvAACT1 in iron translocation The similar expression level of HvAACT1 in the central cylinder tissues of the mature root zone of both cultivars suggests that HvAACT1 has other functions ( Fig. 3g ). HvAACT1 is a homologue of OsFRDL1 in rice and AtFRD3 in Arabidopsis [21] , [22] , which are localized in the pericycle cells and involved in the translocation of iron from the roots to the shoots by transporting citrate into the xylem. To test whether HvAACT1 is also involved in iron translocation, we introduced the Morex-type HvAACT1 into the rice mutant osfrdl1 defective in the translocation of iron [21] . When the mutant was grown at a low Fe concentration (0.2 μM), the new leaves of osfrdl1 mutant showed chlorosis typical of Fe deficiency ( Fig. 5a ), whereas the transgenic lines carrying HvAACT1 rescued the phenotype of the mutant. The SPAD (indicator of chlorophyll content) value of the youngest expanded leaf was lower in the osfrdl1 mutant than the wild-type rice; this was restored to the wild-type level by the transformation with HvAACT1 ( Fig. 5b ). In the presence of high Fe (10 μM), all lines showed similar SPAD values ( Fig. 5c ). 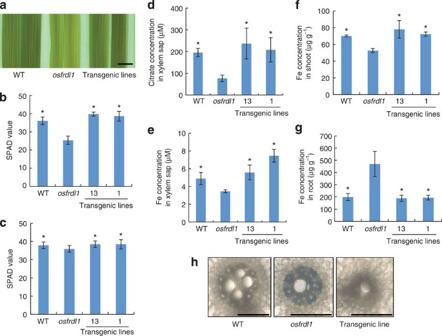Figure 5: Complementation test for iron translocation in rice. (a) Rescue of leaf chlorosis by the introduction of MorexHvAACT1. (b,c) SPAD value of the youngest expanded leaf of transgenic rice carrying Morex-typeHvAACT1promoter grown in a nutrient solution containing 0.2 (b) or 10 (c) μM FeSO4. Data are shown as means±s.d. (n=4–6). (d,e) Concentration of citrate (d) and iron (e) in the xylem sap of different rice lines. (f,g) Concentration of iron in the shoots (f) and roots (g). Data are shown as means±s.d. (n=3–5). Statistical comparison was performed by one-way ANOVA followed by Dunnett's multiple comparison test. *P<0.05. All data were compared withosfrdl1. (h) Rescue of iron precipitation in the roots by the introduction of MorexHvAACT1. Scale bars inaandhindicate 10 mm and 100 μm, respectively. Figure 5: Complementation test for iron translocation in rice. ( a ) Rescue of leaf chlorosis by the introduction of Morex HvAACT1 . ( b , c ) SPAD value of the youngest expanded leaf of transgenic rice carrying Morex-type HvAACT1 promoter grown in a nutrient solution containing 0.2 ( b ) or 10 ( c ) μM FeSO 4 . Data are shown as means±s.d. ( n =4–6). ( d , e ) Concentration of citrate ( d ) and iron ( e ) in the xylem sap of different rice lines. ( f , g ) Concentration of iron in the shoots ( f ) and roots ( g ). Data are shown as means±s.d. ( n =3–5). Statistical comparison was performed by one-way ANOVA followed by Dunnett's multiple comparison test. * P <0.05. All data were compared with osfrdl1 . ( h ) Rescue of iron precipitation in the roots by the introduction of Morex HvAACT1 . Scale bars in a and h indicate 10 mm and 100 μm, respectively. Full size image In the transgenic lines, the concentrations of citrate and iron in the xylem sap were significantly higher than those of the osfrdl1 mutant and were comparable to those of the wild-type rice ( Fig. 5d,e ). Expression of HvAACT1 also increased the iron concentration in the shoots, but decreased the iron concentration in the roots ( Fig. 5f,g ). There were Fe precipitates in the osfrdl1 mutant roots; these disappeared in the transgenic lines ( Fig. 5h ). These results indicate that HvAACT1 also has a role in transporting Fe from the roots to the shoots by releasing citrate to the xylem. Evolutional analysis of HvAACT1 To examine the evolutionary origin of the 1-kb upstream insertion, we investigated its presence in 154 and 265 accessions of wild barley ( Hordeum vulgare ssp. spontaneum ) and cultivated barley ( Hordeum vulgare ssp. vulgare ), respectively, which have been collected from different geographic locations around the world. The insertion was not found in any of the wild barley accessions examined ( Table 1 ). It was detected only in 20 cultivated barley accessions distributed in the acid soil areas in Japan, Korea and China ( Table 1 , Supplementary Fig. S4 ). We compared the Al tolerance of these accessions with 20 other accessions randomly selected from the collection by Eriochrome cyanine staining method, which reflects Al accumulation in the roots ( Supplementary Fig. S5 ). All cultivars with the insertion showed higher Al tolerance (less Al staining) compared with those without the insertion. Table 1 Detection of the 1-kb insertion in HvAACT1 upstream region in wild and cultivated barley. Full size table In order to address the origin and the spread of the 1-kb insertion in the global barley population in more detail, we performed a haploytpe analysis by sequencing the region spanning 1,237 bp within the HvAACT1 gene in 48 barley accessions ( Supplementary Table S1 ). There were only nine single-nucleotide polymorphism and three Indel sites (including the 1-kb insertion) in this region among the accessions tested ( Supplementary Table S2 ). Ten haplotypes can be defined based on the polymorphisms ( Supplementary Table S2 ). Based on the silent base substitutions, we estimated that the nucleotide diversity, π, of the silent sites in the HvAACT1 gene to be 0.0024 and 0.0007 in wild and cultivated barley, respectively. A haplotype network was constructed to examine whether the 1-kb insertion is of single or multiple origins ( Fig. 6 ). The accessions with the 1-kb insertion belong to the haplotype 10, which originated from the haplotype 1 ( Supplementary Fig. S6 ). The relationship between haplotype 10 (with insertion) and haplotype 1 (without insertion) is also supported by the phylogeny of substitution mutations ( Supplementary Fig. S6 ) derived from the Supplementary Table S2 . These results indicate that the 1-kb insertion is from a single origin during the expansion of barley cultivation onto the acid soil areas. 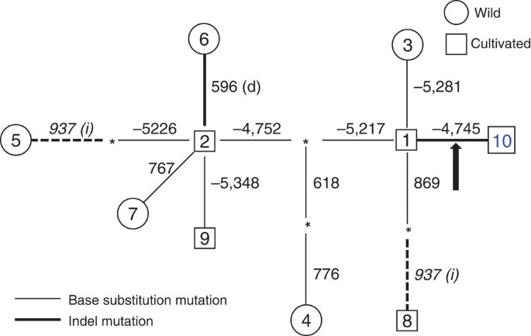Figure 6: Haplotype network among ten haplotypes ofHvAACT1. Haplotype network is constructed using both substitution and Indel polymorphisms by the maximum-parsimony criterion (heuristic search) in PAUP*. Thin and bold lines represent base substitution and Indel mutations, respectively. Asterisks indicate inferred intermediate haplotypes. Numbers above or next to the lines indicate the variable position. A 1-kb insertion in the 5′-flanking region is marked by an arrow. One homoplasious 1-bp insertion is marked by dotted lines. Observed haplotypes in wild barley are shown in circles, and in cultivated barley in squares. Figure 6: Haplotype network among ten haplotypes of HvAACT1 . Haplotype network is constructed using both substitution and Indel polymorphisms by the maximum-parsimony criterion (heuristic search) in PAUP*. Thin and bold lines represent base substitution and Indel mutations, respectively. Asterisks indicate inferred intermediate haplotypes. Numbers above or next to the lines indicate the variable position. A 1-kb insertion in the 5′-flanking region is marked by an arrow. One homoplasious 1-bp insertion is marked by dotted lines. Observed haplotypes in wild barley are shown in circles, and in cultivated barley in squares. Full size image Barley was domesticated from its wild ancestral form H. vulgare ssp. sponatneum in the Near-East about 10,000 years ago [23] . Soils in this region are predominantly alkaline, where there is no threat of Al toxicity stress, whereas the Fe availability is limited. Therefore, barley has developed an efficient strategy for acquiring insoluble iron in alkaline soil by synthesizing and secreting large amount of phytosiderophores [2] . Around 3,000 years ago barley cultivation was expanded to East Asia, where the crop started to encounter Al toxicity stress on acid soils. Our results indicate that cultivated barley acquired Al tolerance through a 1-kb insertion in the upstream of an Al-tolerant gene, HvAACT1 . HvAACT1 encodes a citrate transporter [14] . Its original role in barley is to release citrate to the xylem for efficient translocation of Fe ( Fig. 7 ). Citrate forms complexes with iron in the xylem to prevent Fe precipitation [21] , [22] . The release of citrate to the xylem is mediated by citrate transporters such as AtFRD3 in Arabidopsis [22] and OsFRDL1 in rice [21] ; the barley HvAACT1 is also a homologue of these citrate transporters. They are expressed in the pericycle cells in the mature root zones, where xylem is well developed. When HvAACT1 was introduced into the rice mutant osfrdl1 , it restored all mutant phenotypes, including the concentrations of citrate and Fe in the xylem sap, the leaf chlorophyll content and Fe precipitation in the roots, to the wild-type levels ( Fig. 5 ). Therefore, HvAACT1 in the root pericycle cells functions as a citrate transporter required for the Fe nutrition; this role is conserved in all barley accessions regardless of their Al tolerance ( Figs 3 and 7 ). In fact, HvAACT1 also showed a transport activity for citrate in the absence of Al although the activity was greatly enhanced by Al exposure [14] . 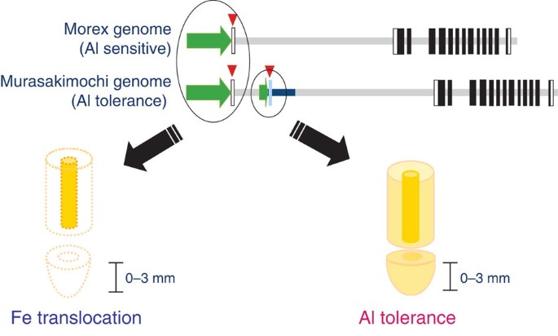Figure 7: Schematic presentation ofHvAACT1roles in barley. HvAACT1 in the pericycle cells of root mature zone releases citrate to the xylem, which is required for the translocation of Fe from the roots to the shoots in both Al-sensitive and -tolerant cultivars. A 1-kb insertion in the upstream in the Al-tolerant cultivars alters the expression to the root tips and enhances the expression in both the root tips and mature zones.HvAACT1expressed in the root tips releases citrate to the rhizosphere to detoxify Al. Figure 7: Schematic presentation of HvAACT1 roles in barley. HvAACT1 in the pericycle cells of root mature zone releases citrate to the xylem, which is required for the translocation of Fe from the roots to the shoots in both Al-sensitive and -tolerant cultivars. A 1-kb insertion in the upstream in the Al-tolerant cultivars alters the expression to the root tips and enhances the expression in both the root tips and mature zones. HvAACT1 expressed in the root tips releases citrate to the rhizosphere to detoxify Al. Full size image Interestingly, HvAACT1 gains a second function with the 1-kb insertion in the upstream of the coding region in the Al-tolerant barley cultivars ( Fig. 7 ). This insertion functions as a promoter because of the presence of multiple transcriptional start sites ( Figs 1 and 2 ). The insertion not only enhances the expression of HvAACT1 in the whole root, but also spatially alters its expression pattern by markedly increasing the expression in the root tips of the Al-tolerant cultivars ( Fig. 3 ). Root tips are the most sensitive target of Al toxicity [24] . The enhanced expression of HvAACT1 in this root zone results in increased citrate secretion to the rhizosphere, thereby protecting the root tips from Al toxicity ( Fig. 4 ). Gene expression is regulated by different mechanisms, such as chromatin condensation, DNA methylation, transcriptional initiation, alternative splicing of RNA, mRNA stability and so on [25] . Among the Al-tolerant genes identified, a minimum MITE insertion size in the promoter region of SbMATE in sorghum was suggested to be involved in regulating the expression of this gene [15] . On the other hand, tandemly repeated elements of length 33–803 bp and located in the upstream of the TaALMT1 -coding region are associated with a high expression of TaALMT1 in wheat [26] , [27] . The mechanism for regulating HvAACT1 expression in barley appears to be distinct from those in other plant species. Furthermore, TaALMT1 and SbMATE are responsible for Al tolerance only, whereas HvAACT1 has evolved dual functions; Fe translocation and Al tolerance. The cultivated accessions of barley are genetically divided into the Western and Eastern groups [28] . The occurrence of the 1-kb insertion in the upstream region of HvAACT1 gene might originate in the Eastern region where acid soils are distributed ( Table 1 ). This is supported by the low nucleotide diversity, π, of HvAACT1 , which is markedly lower than those reported previously for other genes [28] . The low nucleotide diversity of HvAACT1 gene indicates that it is functionally and evolutionally conserved in barley species and that the 1-kb insertion happened during the expansion of barley cultivation into the acid soil areas. This is reasonable considering that the original role of HvAACT1 is to facilitate the translocation of iron. Our study provides evidence for the acquisition of Al tolerance as one of the adaptive traits; it is this adaptation that allows the expansion of barley cultivation onto the acidic soils in the Far-Eastern region. Plant materials and growth conditions Barley ( Hordeum vulgare ) seeds were soaked in deionized water overnight at 20 °C in the dark and then transferred to nets floating on a 0.5 mM CaCl 2 solution in a 1.5-liter plastic container. After growth at 20 °C for 3–4 days, the seedlings were transferred to a 3.5-liter plastic pot containing one-fifth Hoagland solution. Genomic sequence analysis A BAC clone containing HvAACT1 was screened by using primers: 5′-TGGAGGAAGCATAGTATC-3′ and 5′-CACCTGGAGGTATGAA-3′. The shotgun library of the selected BAC was sequenced and assembled to obtain the genomic DNA sequence of HvAACT1 . The upstream of the HvAACT1 genome sequence was obtained from an Al-sensitive cultivar (Morex) and an Al-tolerant cultivar (Murasakimochi) by PCR using primers; 5′-AACAGCTCTGCACCCAGTCGCCGGCCACTT-3′ and 5′-GATGTTCATGACAAAGAGGTAGAG-3′. The fragments obtained were directly sequenced using BigDye Terminators V3.1 cycle sequencing kit on an ABI PRISM 310 genetic analyser. To examine the presence of the insertion in other accessions, 13 accessions differing in Al tolerance, including Morex and Murasakimochi, were used. Fragments including the insertion were amplified by PCR using Takara Ex Taq (Takara) from the genomic DNA extracted from each cultivar. The primers used were 5′-GGTCCAACACTCTACCCTTCCTT-3′ and 5′-GGTGCGAGTTGCCCCTAGCTATTACAGA-3′. The PCR products were separated by electrophoresis on a 1.0% agarose gel using 0.5× TBE buffer stained with ethidium bromide. Identification of the TSS To determine the TSS of HvAACT1 , total RNA from the roots of both Morex and Murasakimochi was isolated with an RNeasy plant Mini Kit (Qiagen). 5′-RACE was performed by GeneRacer kit (Invitrogen) using 2 μg total RNA. The ligated mRNA with RNA oligo adapter was transferred to a first-strand cDNA using SuperScript III RT and the random primers in the reverse-transcription reaction. The 5′ ends of HvAACT1 cDNA were amplified by PCR with the GeneRacer 5′ primer and gene-specific primer 5′-CTCTACCTCTTTGTCATGAACATC-3′, GeneRacer 5′ Nested primer and gene-specific primer 5′-GATGTTCATGACAAAGAGGTAGAG-3′. The PCR products were cloned into pCR2.1 TOPO vector (Invitrogen) and cloned plasmids were sequenced. Transient promoter activity assay To investigate the promoter activity, two different regions were fused with GFP. Putative promoter 1 was located at 1 kb from just after the common TSS, which was amplified by KOD-Plus (Toyobo) using the forward primer, 5′-ACGGACACCTTCGGAGATACCTGTAGAGCA-3′ and reverse primer, 5′-CGCCTATTTATAGGGGCCACACGACCCACCATGG-3′. Putative promoter 2 (262 bp) was located in the specific insertion region just after the most TSS and was amplified using the forward primer, 5′-ATATGCCGTGGACAGAATACAGTTATGCCC-3′ and reverse primer, 5′-CCATGGCCTGGAGTAGGTTGTCTCTCGATGCAGCG-3′. The fragment amplified was introduced into pGEM vector by pGEM-T (Easy) Vector Systems (Promega). These fragments were introduced into the GFP-nopaline synthase (NOS) terminator plasmid, which has the native promoter deleted. As a positive control, GFP was fused to the 35S promoter. The constructs were then bombarded into onion epidermal cells. After overnight incubation, GFP fluorescence was observed with a confocal laser scanning microscopy (LSM700; Carl Zeiss). Expression pattern analysis Roots of both Morex and Murasakimochi grown in a 0.5-mM CaCl 2 solution for 4 days were separated into different segments (0–3, 3–6, 6–9, 9–12, 12–20 mm) with a razor. The samples were ground in liquid nitrogen and total RNA was isolated with RNeasy plant Mini Kit (Qiagen). cDNA was synthesized as described above. The expression levels of HvAACT1 in different root zones were quantified by absolute quantitative real-time PCR using different primers. For the common UTR region, primers used were 5′-GCCAGTAGCTCTCTGCGCTC-3′ and 5′-CCTGAAGTGGCGAAGTGG-3′. For the specific insertion region, primers used were 5′-GCTGCATCGAGAGACAACCT-3′ and 5′- TCAGAAGCTGTCTGCTCGGG-3′, and for the coding region, the following primers were used: 5′-TTCGTCGCTGAAGAAGATGC-3′ and 5′-GCACATTGCAGGCATCTGAA-3′. Reactions were run on the MasterCycler ep realplex (Eppendorf). To generate standard curves for absolute quantification for each region, a series of dilutions (from 1×10 −1 to 10 −6 ng) of plasmids were made and then assayed by real-time PCR. C T values for each sample were converted into absolute copy numbers using the standard curves. To investigate tissue-specific expression of HvAACT1 , laser microdissection was performed by the method of Takahashi et al . [29] Roots of both Morex and Murasakimochi were dissected at 0.5–3.5 mm and 18.5–21.5 mm to collect anteroposterior 1.5 mm in a surplus. The samples were immediately immersed in a fixing solution containing ethanol/acetic acid at a 3:2 ratio. Central cylinder and outer tissues were collected from the root tissue sections using a Veritas Laser Microdissection System LCC1704 (Molecular Devices) and used for total RNA extraction. The cDNA from each sample was used for the quantitative analysis of gene expression. Cyclophilin was used as an internal control by the ΔΔCt method. HvAACT1 expression levels were normalized with that in the 0–3 mm central cylinder of Morex. Preparation of transgenic barley and rice The promoter region was amplified by 5′-GGTACCACGGACACCTTCGGAGATACCT-3′ and 5′-GGACGTCGACGACGGCCACCCACTTCTTGT-3′ primers for the B1 fragment, 5′-TACCTGCAGGCAGTAGCTCTCTGCGCTCAG-3′ and 5′-GGACGTCGACGACGGCCACCCACTTCTTGT-3′ primers for the B3 fragment from Murasakimochi genomic DNA, using KOD-FX (Toyobo; Supplementary Figs S1 and S6 ). The B2 promoter region was amplified by 5′-GGTACCACGGACACCTTCGGAGATACCT-3′ and 5′-ACAAGAAGTGGGTGGCCGTCGTCGACGTCC-3′ primers from the Morex genomic DNA ( Supplementary Figs S1 and S6 ). These fragments were cloned into pCR2 vector by TOPO XL PCR Kit (Invitrogen). The HvAACT1 open reading frame (ORF) was amplified by using forward primer 5′-ACTCCTCTGTCCGAGCACGA-3′ and reverse primer 5′-CCCGGGCTCCTCGCACAAAAGGCAGACGACC-3′ by using KOD-FX from the Morex cDNA. This fragment was cloned into pGEM vector (Promega) and sequenced. The ORF was inserted between with NOS terminator into pUC19 vector. The plasmids of cloned promoters as described above were digested by Kpn I and Bam HI and the plasmid of cloned ORF-NOS terminator was digested by Not I and Bam HI. These fragments were ligated into pPZP vector [30] and then transformed into Agrobacterium tumefaciens (strain EHA101). Immature embryos of barley cultivar Golden Promise were used for Agrobacterium-mediated transformation [31] , [32] , [33] . We obtained several independent transgenic lines and three or four each were randomly selected for further analysis. Transformation of the Morex promoters fused with HvAACT1 cDNA into a rice mutant osfrdl1 defective in iron translocation [21] was performed [34] . Phenotypic analysis of transgenic barley and rice To measure Al tolerance, transgenic barley lines were exposed to a 1-mM CaCl 2 solution with or without 3 μM Al at pH 5.0. Root elongation during 24 h was measured with a ruler. Root exudates of the transgenic lines and WT (3 weeks old) were collected by exposing plants to a 1-mM CaCl 2 solution containing 10 μM Al for 6 h. Citrate was measured by an enzymatic method [35] . Transgenic rice lines, WT and osfrdl1 mutant were grown in a one-half strength Kimura B solution containing 0.2 μM or 10 μM FeSO 4 at 25 °C. The SPAD value of the youngest fully expanded leaf was measured after growth for 15 days. Plants grown in the presence of 0.2 μM FeSO 4 were decapitated at 2 cm above the roots and the xylem sap was collected from the cut end for 1 h by micropipette. The concentrations of citrate and iron in the xylem sap were determined as described previously [21] . The Fe concentrations in the roots and shoots were determined by ICP-MS (Aglient Technologies). Perls' staining was performed in plants grown in a solution containing 10 μM FeSO 4 for 1 month [21] . Geographic distribution analysis A total of 265 cultivated barley accessions collected from around the world and 154 wild barley accessions were used to examine the presence of the specific insertion. Primers for amplified fragments including the insertion region were used. Genomic DNA was extracted from each accession and used as a template. Touchdown PCR was run by using KOD-FX, followed by standard PCR performed after 30 cycles. Al tolerance was evaluated by Eriochrome cyanine staining [36] . A total of 40 cultivars including 20 with the insertion and 20 without the insertion, which were randomly selected from the collection, were used. Seedlings (1-week-old) were exposed to a 1.0-mM CaCl 2 solution (pH 5.0) for 48 h and then stained in 0.1% Eriochrome cyanine for 15 min [36] . Roots were then washed with deionized water and photographed. The distribution of barley accessions with or without the insertion was mapped onto a world soil atlas with different soil pHs ( http://www.sage.wisc.edu/atlas/maps.php?datasetid=20&includerelatedlinks=1&dataset=20 ). The information of the accession origin of cultivated barley was based on Barley DB ( http://www.shigen.nig.ac.jp/barley/collectionMap/map.html ). Wild barley accessions have been described by Konishi [37] ( Supplementary Table S3 ). Phylogenic analysis To generate a neighbour-joining tree, we sequenced the region spanning 1,237 bp within the HvAACT1 gene (688 bp from flanking region to the insertion and 549 bp from the second intron) in 48 barley accessions comprising of 40 cultivated ones and 8 wild ancestors, H. spontaneum ( Supplementary Table S1 ). Alignment of all sequences was performed by ClustalW. Regions containing gaps and missing data were not included. Neighbour-joining tree was constructed with MEGA5. The evolutionary distances were computed using the Kimura 2-parameter method. Bootstrap test with 1,000 replicates was also carried out by MEGA5. Haplotype network analysis Haplotype network was constructed using both substitution and Indel polymorphisms by the maximum-parsimony criterion (heuristic search) in PAUP* (ref. 38 ). Indel mutations were recoded and treated as a fifth base, and all the Indel sites were considered as a single mutation. Accession codes: The nucleotide sequence data reported in this paper has been deposited in the DDBJ/EMBL/GenBank nucleotide sequence databases under the accession numbers AB302223 (cDNA) and AB331641 (genomic DNA). How to cite this article: Fujii, M. et al . Acquisition of aluminium tolerance by modification of a single gene in barley. Nat. Commun. 3:713 doi: 10.1038/ncomms1726 (2012).